Distant residues mediate picomolar binding affinity of a protein cofactor Numerous proteins require cofactors to be active. Computer simulations suggest that cooperative interaction networks achieve optimal cofactor binding. There is a need for the experimental identification of the residues crucial for stabilizing these networks and thus for cofactor binding. Here we investigate the electron transporter flavodoxin, which contains flavin mononucleotide as non-covalently bound cofactor. We show that after binding flavin mononucleotide with nanomolar affinity, the protein relaxes extremely slowly (time constant ~5 days) to an energetically more favourable state with picomolar-binding affinity. Rare small-scale openings of this state are revealed through H/D exchange of N(3)H of flavin. We find that H/D exchange can pinpoint amino acids that cause tight cofactor binding. These hitherto unknown residues are dispersed throughout the structure, and many are located distantly from the flavin and seem irrelevant to flavodoxin's function. Quantification of the thermodynamics of ligand binding is important for understanding, engineering, designing and evolving ligand-binding proteins. Many proteins bind ligands, which usually contact a rather limited number of amino-acid residues. However, their binding effects can propagate to residues that have no direct interaction with the ligand and as a result enable biological phenomena such as allosteric regulation and signal transduction [1] , [2] . During binding, a ligand selects the protein conformers that best match its structural and dynamic properties among the pool of conformers intrinsically accessible to the protein in unliganded form [3] . Cofactors form a special category of ligands. A cofactor is a non-protein chemical compound that is bound to a protein and is required for the protein's biological activity. On binding, the properties of both cofactor and protein can mutually alter, as happens, for instance, in case of hemo- or flavoproteins, thereby facilitating important life processes like electron transfer. Dynamic fluctuations are fundamentally linked to protein function. Fluorescence and nuclear magnetic resonance (NMR) spectroscopy have illuminated fast internal protein dynamics and their biological purpose. For example, NMR relaxation methodologies, which reveal protein dynamics on the millisecond timescale and below, enable characterization of dynamic features of enzymes relevant for catalysis [4] , [5] . On ligand binding, significant changes in fast internal dynamics can occur. This perturbation might be local, or transmitted to sites remote from the binding site [6] . Usually, binding of a ligand reduces protein flexibility. However, nature sometimes employs increases in the residual entropy of proteins, manifested in their conformational dynamics, as a thermodynamic mechanism for allosteric responses to ligand binding. Hence, enhanced internal protein dynamics on ligand binding have been observed as well [7] , [8] . Computer simulations suggest that propagation of ligand-binding interactions and protein stability are linked. This link is mediated through distribution of stability within different structural elements of a protein, and interactions existing between them [9] . By means of these interaction networks, ligand-induced stabilization can transmit throughout a protein. Although considerable progress has been made in computational studies of ligand binding [10] , [11] , [12] , [13] , a strong need exists for experimental data that probe and verify, at the residue level, the effects ligand binding have on protein thermodynamic stability. Flavoproteins are cofactor-containing proteins that participate in various biological functions, such as photosynthesis, cellular respiration, DNA repair, apoptosis, and nerve signal transmission [14] . Flavodoxins are monomeric electron transfer proteins and contain flavin mononucleotide (FMN) that can exist as oxidized quinone, one electron-reduced semiquinone and two-electron reduced hydroquinone [15] , [16] . The redox potentials of flavodoxins are affected by several factors, including a conserved tyrosine that tightly packs onto the isoalloxazine ring of FMN and differentially interacts with it on changing redox states, stabilization of the semiquinone relative to the oxidized form (because it forms a new hydrogen bond with a main chain group), repelling interactions of the negatively charged isoalloxazine ring of two-electron-reduced FMN with both acidic residues on the periphery of the protein and the negatively charged phosphate of FMN, and unfavourable burial inside the hydrophobic interior of flavodoxin of this uncompensated negative charge [16] , [17] , [18] . As a result, flavodoxin can transfer electrons between various physiological redox partners. Strong binding of FMN is essential for flavodoxins to be functionally active, and these proteins are remarkably rigid on the ns-timescale and below [19] , [20] , [21] , [22] . The isoalloxazine moiety and 5′-phosphate group of FMN contribute almost equally to the free energy associated with cofactor binding, whereas the ribityl has barely any impact [23] . Currently, amino-acid residues crucial for stabilizing FMN–protein interactions are unknown. Thus, whereas the redox potential-affecting contributions of flavodoxin have been revealed, the structural determinants that govern strong cofactor binding are still obscure. Use of H/D exchange detected by NMR spectroscopy can identify amino-acid residues that are required for tight cofactor binding. Because of an unfolding process, a residue can arrive in an open or exchange-competent form from which amide proton exchange with deuterons takes place when a protein is dissolved in deuterium oxide. For some residues, the dominant process that causes amide exchange to occur is a highly local opening of the native protein structure. For other residues, exchange only happens if rare opening events like subglobal or global protein unfolding occur. These unfolding processes typically occur on timescales ranging from seconds to many days [24] , [25] . Using H/D exchange data, thermodynamic stabilities against unfolding can be quantified, leading to first efforts to address the influences ligand binding has on local protein stabilities (see example in refs 26 , 27 , 28 , 29 ). To correctly interpret H/D exchange data of a cofactor-containing protein, knowledge about the (un)folding and local thermodynamic stabilities of the corresponding apoprotein is required, as well as a thorough understanding of the role cofactor binding has in protein folding. We demonstrated that the in vitro folding of apoflavodoxin (that is, flavodoxin without FMN) occurs autonomously and spontaneously and involves two intermediates [30] , [31] , [32] , [33] . Non-covalent binding of FMN to native apoflavodoxin is the last step in flavodoxin folding, and during global unfolding of flavodoxin, release of FMN happens first [31] . NMR data showed that native apoflavodoxin strongly resembles flavodoxin, except for dynamic disorder in the flavin-binding region [34] . Here we report the effects cofactor binding has on local thermodynamic stabilities of a flavodoxin from Azotobacter vinelandii . We demonstrate that after reconstitution from apoprotein and FMN, flavodoxin relaxes extremely slowly to an energetically more favourable state with two orders of magnitude better FMN binding. We apply H/D exchange to investigate local thermodynamic stabilities of relaxed flavodoxin, which has picomolar binding affinity for FMN. We show that N(3)H of flavin is an excellent probe to follow opening events in flavin-binding sites and identify amino-acid residues that cause tight binding of the cofactor. Determination of the strength of FMN binding We determined the equilibrium constant for dissociation of FMN from flavodoxin (that is, K D ) according to a well-established procedure in which aliquots of apoprotein are titrated to an FMN solution ( Supplementary Methods ). Use is made of the severe quenching of the fluorescence of FMN on its binding to apoprotein [31] , [35] . Quenching happens within seconds [31] . After each addition of apoprotein, the system was allowed to equilibrate for 5 min in the dark before recording of FMN fluorescence ( Fig. 1a ). We derive that K D is (3.51±0.20)·10 −10 M, which is fully consistent with K D -values reported for other flavodoxins [36] . 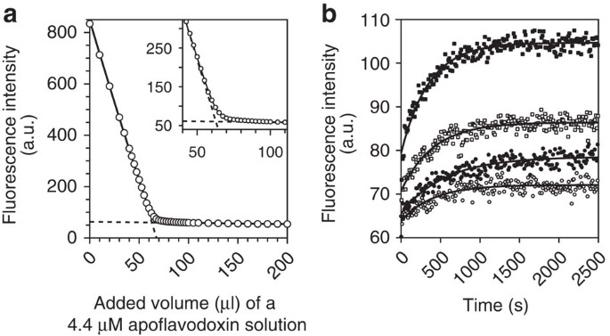Figure 1: Equilibrium constant for dissociation of FMN from flavodoxin and corresponding rate constant. (a) Determination ofKDusing the quenching of FMN fluorescence on binding of this cofactor to apoprotein at 25 °C. A 188-nM FMN solution is titrated with aliquots of a 4.4-μM apoflavodoxin solution. One unit of fluorescence corresponds to 0.22 nM FMN. Equation (S8) ofSupplementary Methodsis fitted to the resulting fluorescence intensity data andKDis determined to be (3.51±0.20)·10−10M. The two linear components of this equation are shown as dashed lines. The inset highlights the curved part of the titration data. (b) On dilution of flavodoxin in buffer at 25 °C, FMN is released and fluorescence increases accordingly (fluorescence emission of FMN is followed at 525 nm, while excitation occurred at 450 nm). One unit of fluorescence corresponds to 5.0 nM FMN. After dilution of 5 (open circles), 10 (closed circles), 20 (open squares) and 50 (closed squares) μl of 362 μM flavodoxin in 2,000 μl buffer, respectively, reestablishment of the equilibrium between apo- and holoprotein proceeds exponentially as function of time. Equation (S11) ofSupplementary Methodsis globally fitted to the four relaxation traces and shows thatkoffis (1.05±0.04)·10−6s−1andKDis (3.82±0.12)·10−12M. Figure 1: Equilibrium constant for dissociation of FMN from flavodoxin and corresponding rate constant. ( a ) Determination of K D using the quenching of FMN fluorescence on binding of this cofactor to apoprotein at 25 °C. A 188-nM FMN solution is titrated with aliquots of a 4.4-μM apoflavodoxin solution. One unit of fluorescence corresponds to 0.22 nM FMN. Equation (S8) of Supplementary Methods is fitted to the resulting fluorescence intensity data and K D is determined to be (3.51±0.20)·10 −10 M. The two linear components of this equation are shown as dashed lines. The inset highlights the curved part of the titration data. ( b ) On dilution of flavodoxin in buffer at 25 °C, FMN is released and fluorescence increases accordingly (fluorescence emission of FMN is followed at 525 nm, while excitation occurred at 450 nm). One unit of fluorescence corresponds to 5.0 nM FMN. After dilution of 5 (open circles), 10 (closed circles), 20 (open squares) and 50 (closed squares) μl of 362 μM flavodoxin in 2,000 μl buffer, respectively, reestablishment of the equilibrium between apo- and holoprotein proceeds exponentially as function of time. Equation (S11) of Supplementary Methods is globally fitted to the four relaxation traces and shows that k off is (1.05±0.04)·10 −6 s −1 and K D is (3.82±0.12)·10 −12 M. Full size image To quantify the rate constant for FMN release, k off , we followed the increase in flavin fluorescence due to cofactor dissociation after dilution of flavodoxin in buffer. Reestablishment of equilibrium between apo- and holo-protein proceeds mono-exponentially as function of time, allowing determination of k off , as well as K D ( Supplementary Methods ) [37] . Figure 1b reports four relaxation traces as well as the global fit of equation (S11) of Supplementary Methods to the data. We thus derive that k off is (1.05±0.04)·10 −6 s −1 . Remarkably, now K D is established to be (3.82±0.12)·10 −12 M; that is, FMN binds two orders of magnitude better to apoprotein than the titration procedure reports. Fluorescence spectroscopy is used to elucidate the source for the difference in K D observed. Fluorescence of 5 μM flavodoxin shows a peak at 525 nm characteristic for free FMN ( Fig. 2a ), which is dissociated from holoprotein as K D dictates. On adding excess apoprotein, free FMN is no longer detected. In case of 5 μM reconstituted flavodoxin, obtained by mixing apoflavodoxin and FMN at equimolar ratio higher FMN fluorescence is observed. On adding excess apoprotein a peak is detected at 512 nm ( Fig. 2a ). This 13 nm blue-shifted fluorescence cannot be due to free flavin, but must arise from FMN bound to reconstituted flavodoxin. Clearly, reconstituted protein differs from flavodoxin, explaining the difference in K D -values observed. Inspection of FMN fluorescence of reconstituted flavodoxin reveals that disappearance of fluorescence proceeds extremely slowly with time on relaxation of holoprotein ( Fig. 2b ). 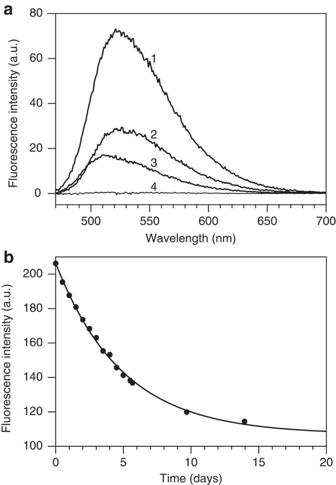Figure 2: Fluorescence emission of flavodoxin and of reconstituted holoprotein. (a) Spectrum-2 is of 5 μM flavodoxin in buffer, whereas spectrum-1 is of 5 μM reconstituted flavodoxin, which is obtained by mixing apoflavodoxin and FMN at equimolar ratio. On subsequent addition of excess apoflavodoxin to a final concentration of 375 nM, fluorescence emission of both samples changes differently (spectrum-4 and spectrum-3, respectively). This addition reveals that fluorescence of FMN in flavodoxin is fully quenched, whereas in freshly reconstituted holoprotein, it is not. (b) Time-dependent change in fluorescence emission of 5 μM reconstituted flavodoxin (excitation 450 nm, emission 514 nm). One unit of fluorescence corresponds to 0.88 nM FMN. Single-exponential fitting of the data shows that the relaxation time is 4.9±0.2 days. Figure 2: Fluorescence emission of flavodoxin and of reconstituted holoprotein. ( a ) Spectrum-2 is of 5 μM flavodoxin in buffer, whereas spectrum-1 is of 5 μM reconstituted flavodoxin, which is obtained by mixing apoflavodoxin and FMN at equimolar ratio. On subsequent addition of excess apoflavodoxin to a final concentration of 375 nM, fluorescence emission of both samples changes differently (spectrum-4 and spectrum-3, respectively). This addition reveals that fluorescence of FMN in flavodoxin is fully quenched, whereas in freshly reconstituted holoprotein, it is not. ( b ) Time-dependent change in fluorescence emission of 5 μM reconstituted flavodoxin (excitation 450 nm, emission 514 nm). One unit of fluorescence corresponds to 0.88 nM FMN. Single-exponential fitting of the data shows that the relaxation time is 4.9±0.2 days. Full size image When freshly reconstituted flavodoxin is subjected to a quick cycle of two-electron reduction and immediate re-oxidation, we detect full quenching of FMN fluorescence, which is the hallmark of relaxed flavodoxin. This observation reveals that tightening of cofactor binding can happen rapidly. On reduction of flavodoxin, N(5) of the flavin becomes protonated. This N(5)H proton forms a hydrogen bond with a specific carbonyl oxygen of the protein backbone, causing the corresponding peptide bond to flip [15] . This redox-modulated conformational change is the most likely source that causes rapid tightening of flavin binding. This rapid tightening is of functional relevance, because flavodoxins act in the reducing environment of the cytoplasm as one-electron carriers by cycling between the semiquinone and hydroquinone forms of FMN. To identify flavodoxin residues involved in slow structural relaxation after cofactor binding, 15 N-labelled apoflavodoxin and 15 N-labelled FMN were mixed. Subsequently, a series of 1 H- 15 N heteronuclear single-quantum coherence (HSQC) spectra was recorded, which reveals that 54 backbone amide cross-peaks of this 179-residue protein shift during a period of 58 days ( Fig. 3 ). 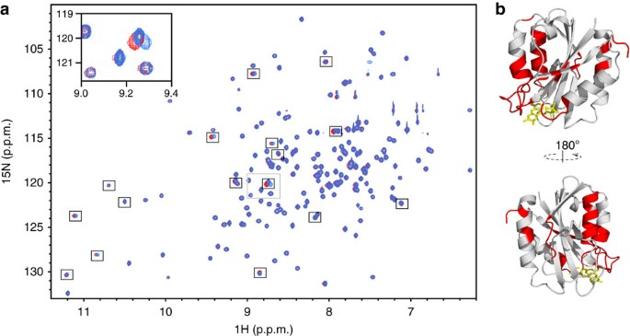Figure 3: Slow structural relaxation within reconstituted flavodoxin. (a) Overlay of1H-15N HSQC spectra recorded 33 min (blue) and 58 days (red) after addition of15N-labelled FMN to15N-labelled apoflavodoxin. Flavodoxin concentration is 2.2 mM in 100 mM potassium pyrophosphate, 90% H2O/10% D2O, pH 6.0, at 25 °C. Cross-peaks that shift prominently are highlighted by black boxes. The inset zooms in on the area that is outlined by a grey box. (b) Amino-acid residues of which the corresponding cross-peaks shift by 0.003 p.p.m. or more are coloured red in the cartoon model of flavodoxin. Figure 3: Slow structural relaxation within reconstituted flavodoxin. ( a ) Overlay of 1 H- 15 N HSQC spectra recorded 33 min (blue) and 58 days (red) after addition of 15 N-labelled FMN to 15 N-labelled apoflavodoxin. Flavodoxin concentration is 2.2 mM in 100 mM potassium pyrophosphate, 90% H 2 O/10% D 2 O, pH 6.0, at 25 °C. Cross-peaks that shift prominently are highlighted by black boxes. The inset zooms in on the area that is outlined by a grey box. ( b ) Amino-acid residues of which the corresponding cross-peaks shift by 0.003 p.p.m. or more are coloured red in the cartoon model of flavodoxin. Full size image Quantification of thermodynamic stabilities To reveal how FMN locally affects the stabilities of flavodoxin's residues against exposure to solvent, we measured H/D exchange rates (that is, k ex ) of backbone amides of apo- as well as of non-reconstituted holo-protein ( Supplementary Table S1 ). Lyophilized 15 N-labelled protein was dissolved into D 2 O containing 100 mM potassium pyrophosphate at 25 °C, pD 6.3. Each sample was transferred immediately into a NMR instrument and subsequently a series of 1 H- 15 N HSQC spectra was recorded. To obtain k ex , we analysed time-dependent maximal cross-peak intensities of backbone amides ( Supplementary Methods ). 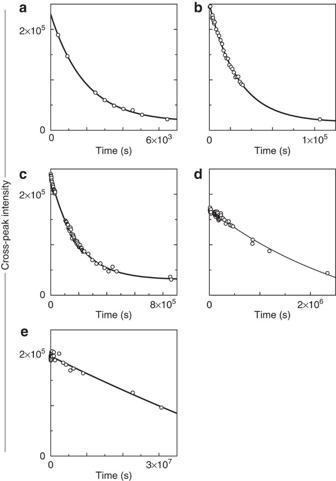Figure 4: Typical H/D exchange curves for backbone amides of flavodoxin. Shown are time-dependent decreases of maximal intensities of cross-peaks arising from backbone amides of (a) Arg24 (kex=(4.12±0.05)·10−4s−1), (b) Ala45 (kex=(3.27±0.02)·10−5s−1), (c) Phe49 (kex=(4.14±0.01)·10−6s−1), (d) Val125 (kex=(5.16±0.04)·10−7s−1) and (e) Leu110 (kex=(2.15±0.03)·10−8s−1), respectively. Notice the hugely different time-scales in panelsa–e. Data are extracted from1H-15N HSQC spectra. Figure 4a–e show typical exchange curves for flavodoxin. Figure 4: Typical H/D exchange curves for backbone amides of flavodoxin. Shown are time-dependent decreases of maximal intensities of cross-peaks arising from backbone amides of ( a ) Arg24 ( k ex =(4.12±0.05)·10 −4 s −1 ), ( b ) Ala45 ( k ex =(3.27±0.02)·10 −5 s −1 ), ( c ) Phe49 ( k ex =(4.14±0.01)·10 −6 s −1 ), ( d ) Val125 ( k ex =(5.16±0.04)·10 −7 s −1 ) and ( e ) Leu110 ( k ex =(2.15±0.03)·10 −8 s −1 ), respectively. Notice the hugely different time-scales in panels a – e . Data are extracted from 1 H- 15 N HSQC spectra. Full size image Quantitative interpretation of H/D exchange is possible using a simple model in which an open or exchange-competent form and a closed or exchange-incompetent form of a protein at the site of a particular amide proton interconvert ( Supplementary Methods ) [38] . Two limiting situations exist in H/D exchange. In case of EX1 exchange behaviour, the exchange rate k ex does not depend on pD and equals the rate constant for local opening of the protein structure, k op . In case of EX2 exchange behaviour, log( k ex ) depends linearly on pD with a slope of 1 and k ex -values can be directly converted into free energy differences between open and closed states, that is, Δ G op -values ( Fig. 5a,b ; Supplementary Methods ). EX2 exchange behaviour has been shown to apply for apoflavodoxin at pD 6.3 (ref. 33 ), and thus we can extract Δ G op -values from the H/D exchange rates of the backbone amides of apoflavodoxin ( Fig. 6a ; Supplementary Table 1 ). To determine the mechanism by which amides of flavodoxin exchange, we measured H/D exchange at pD 6.2, 6.3, 7.7 and 8.8 ( Supplementary Table 2 , 25 °C). The strong pD-dependence of the exchange data collected shows that at pD 6.3, EX2 conditions apply ( Supplementary Methods , and Fig. 5b as example). This observation implies that at this pD, one can directly convert amide exchange rates of flavodoxin into corresponding Δ G op -values ( Fig. 6b ; Supplementary Table S1 ). 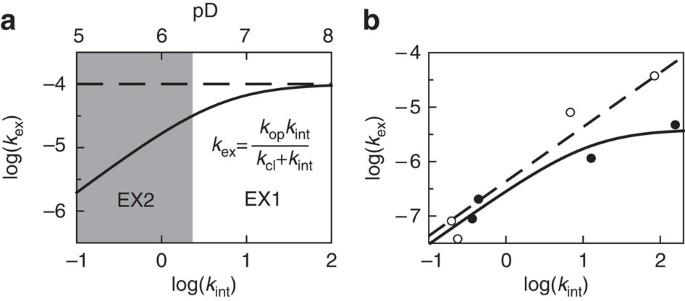Figure 5: pD-dependence of hydrogen exchange. (a) Simulated pD-dependent exchange curve of an exchangeable proton. The intrinsic exchange rate constant,kint, is 1 s−1at pD 6; the rate constant for local opening of the protein,kop, is 1×10−4s−1, and the rate constant for local closing of the protein,kcl, is 5 s−1. An increase of pD by one unit causeskintto increase tenfold. At low pD-values, exchange rate constantkexincreases accordingly (area shaded in grey). In this so-called EX2 pD regime, the logarithm ofkexdepends linearly on pD with a slope of 1. Above a certain pD-value,kintis larger thankcl, and exchange enters the EX1 regime, in whichkexcurves towards a horizontal line defined bykexequallingkop. (b) Measured dependence at 25 °C ofkexonkintof the backbone amides of Leu34 (open circles) and Thr56 (closed circles) of flavodoxin, respectively. Leu34 shows typical EX2 behaviour over the entire pD-range sampled, becausekexincreases tenfold with every increase of pD by one unit. Consequently, ΔGopcan be obtained in this pD-range, because ΔGop=−RTln(kex/kint). When on increasingkint, the value ofkexcurves, as seen here for Thr56, ΔGopcan only be determined at low pD-values, and equation (S4) ofSupplementary Methodscan be fitted to the corresponding data (solid line) to obtainkopandkcl. Figure 5: pD-dependence of hydrogen exchange. ( a ) Simulated pD-dependent exchange curve of an exchangeable proton. The intrinsic exchange rate constant, k int , is 1 s −1 at pD 6; the rate constant for local opening of the protein, k op , is 1×10 −4 s −1 , and the rate constant for local closing of the protein, k cl , is 5 s −1 . An increase of pD by one unit causes k int to increase tenfold. At low pD-values, exchange rate constant k ex increases accordingly (area shaded in grey). In this so-called EX2 pD regime, the logarithm of k ex depends linearly on pD with a slope of 1. Above a certain pD-value, k int is larger than k cl , and exchange enters the EX1 regime, in which k ex curves towards a horizontal line defined by k ex equalling k op . ( b ) Measured dependence at 25 °C of k ex on k int of the backbone amides of Leu34 (open circles) and Thr56 (closed circles) of flavodoxin, respectively. Leu34 shows typical EX2 behaviour over the entire pD-range sampled, because k ex increases tenfold with every increase of pD by one unit. Consequently, Δ G op can be obtained in this pD-range, because Δ G op = −RT ln( k ex / k int ). When on increasing k int , the value of k ex curves, as seen here for Thr56, Δ G op can only be determined at low pD-values, and equation (S4) of Supplementary Methods can be fitted to the corresponding data (solid line) to obtain k op and k cl . 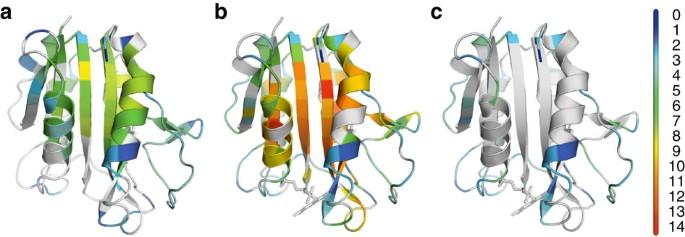Figure 6: Thermodynamic stabilities of apoflavodoxin and flavodoxin. The cartoon models show ΔGopat the residue level of (a) apoflavodoxin and of (b) flavodoxin, as determined by H/D exchange at pD 6.3, 25 °C. Residues are colour-coded according to the scale bar shown, with ΔGop-values in kcal mol−1. Residues for which ΔGop-values could not be determined are shown in grey. (c) Same as (b), but showing only those residues of flavodoxin for which ΔGopis smaller than 5 kcal mol−1. The cartoon models are generated with PyMOL (Schrödinger, LLC, Palo Alto, CA, USA) using the crystal structure ofA. vinelandiiflavodoxin (pdb ID 1YOB48), and the FMN cofactor is shown in stick representation. Full size image Figure 6: Thermodynamic stabilities of apoflavodoxin and flavodoxin. The cartoon models show Δ G op at the residue level of ( a ) apoflavodoxin and of ( b ) flavodoxin, as determined by H/D exchange at pD 6.3, 25 °C. Residues are colour-coded according to the scale bar shown, with Δ G op -values in kcal mol −1 . Residues for which Δ G op -values could not be determined are shown in grey. ( c ) Same as ( b ), but showing only those residues of flavodoxin for which Δ G op is smaller than 5 kcal mol −1 . The cartoon models are generated with PyMOL (Schrödinger, LLC, Palo Alto, CA, USA) using the crystal structure of A. vinelandii flavodoxin (pdb ID 1YOB [48] ), and the FMN cofactor is shown in stick representation. Full size image FMN-induced stabilization varies widely across holoprotein The H/D exchange data set obtained of apo- and holo-protein ( Fig. 4 ; Supplementary Tables S1 and S2 ) allows assessment of the effects FMN binding has on protecting residues against exchange. The term ΔΔ G op =(Δ G op (flavodoxin)−Δ G op (apoflavodoxin)) quantifies the change in stability against exposure to solvent of the residues of apoflavodoxin as a result of FMN binding. For 87 residues of flavodoxin, we obtained ΔΔ G op -values, because the corresponding Δ G op -values of both apo- and holo-protein are available ( Supplementary Table S1 ; the standard deviation of Δ G op is 0.35 kcal mol −1 ( Supplementary Methods ), and consequently, the standard deviation of ΔΔ G op is 0.50 kcal mol −1 ). 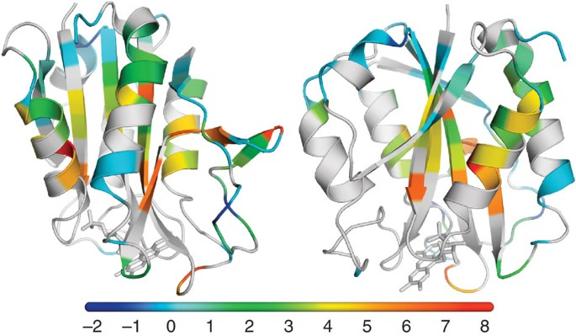Figure 7: Binding of FMN thermodynamically stabilizes flavodoxin. The cartoon models show the differences in ΔGopat the residue level (that is, ΔΔGop) between flavodoxin and apoflavodoxin at pD 6.3, 25 °C. The models are rotated by 90° relative to one another. Residues are colour-coded according to the scale bar shown, with ΔΔGop-values in kcal mol−1. Residues that are not affected on incorporation of FMN (that is, −0.5< ΔΔGop<0.5 kcal mol−1) are coloured pale blue. Residues for which ΔΔGop-values could not be determined are shown in grey. Figure 7 shows that the magnitudes of ΔΔ G op -values vary widely across flavodoxin. These magnitudes do not correlate with Δ G op (apoflavodoxin) ( Supplementary Fig. S1 ). For 30 residues (coloured pale blue in Fig. 7 ), the corresponding ΔΔ G op -values equal within error 0 kcal mol −1 (that is, −0.5<ΔΔ G op <0.5 kcal mol −1 ). These residues reside in parts of the protein where binding of FMN apparently does not affect protein dynamics relevant for H/D exchange. Many of these 30 residues are located within or close to the part of the parallel β-sheet that is opposite to the site where FMN binds, suggesting that the more distant a residue is from FMN, the less stabilized it is. However, no significant correlation between ΔΔ G op and the distance a residue has to FMN exists ( Supplementary Fig. S2 ). Three peripheral residues become less protected against exposure to water on incorporation of FMN (that is, Tyr47, Gly132 and Ser138, coloured dark blue in Fig. 7 ). Significant FMN-induced stabilization of the protein occurs for 54 residues (coloured green, yellow, orange and red in Fig. 7 ), because the corresponding ΔΔ G op -values exceed 0.5 kcal mol −1 ( Supplementary Table S1 ). Figure 7: Binding of FMN thermodynamically stabilizes flavodoxin. The cartoon models show the differences in Δ G op at the residue level (that is, ΔΔ G op ) between flavodoxin and apoflavodoxin at pD 6.3, 25 °C. The models are rotated by 90° relative to one another. Residues are colour-coded according to the scale bar shown, with ΔΔ G op -values in kcal mol −1 . Residues that are not affected on incorporation of FMN (that is, −0.5< ΔΔ G op <0.5 kcal mol −1 ) are coloured pale blue. Residues for which ΔΔ G op -values could not be determined are shown in grey. Full size image H/D exchange reports cofactor-induced protein stabilization Because of bound FMN, the stability against global unfolding of flavodoxin (that is, Δ G N-U ( flavodoxin )) is higher than that of apoflavodoxin. This stability difference depends on the concentration of free FMN [39] : in which R is the gas constant, T the absolute temperature, and [ FMN ] the concentration of free FMN in solution. H/D exchange experiments are done using non-reconstituted flavodoxin with a concentration of about 2.75 mM and consequently, using a K D of (3.82±0.12)·10 − 12 M, the concentration of FMN not bound to protein is 102 nM (that is, binding site saturation is >99.996%). According to equation (1), cofactor binding to apoflavodoxin contributes 6.0 kcal mol −1 to flavodoxin's global stability. One would expect that the residues with the largest ΔΔ G op -values report the magnitude of cofactor-induced stabilization of holoprotein. Indeed, ten residues of flavodoxin show a stability increase compared with apoflavodoxin that equals within error 6.0 kcal mol −1 . Stabilization with 5.0<ΔΔ G op <7.0 kcal mol −1 (that is, 6.0 kcal mol −1 ± twice the s.d. of ΔΔ G op ) happens for Gly8, Ala92, Gly95, Tyr102, Asp143, Phe146, Val147 Gly148, Ala150 and Leu151, which are coloured orange and red in Fig. 7 . Hence, on binding of FMN, these parts of the protein stiffen to such an extent that H/D exchange of the corresponding amides from holoprotein hardly happens. However, on occasional release of FMN, this exchange does occur from apoflavodoxin and is subsequently detected, thereby quantitatively revealing the cofactor-induced stabilization of holoprotein against global unfolding. Most of these ten amino-acid residues, except for Gly8 and Tyr102, are far from the flavin and experience long-range stabilization effects. The ΔΔ G op -value of one residue of flavodoxin is remarkably high (that is, Ala18; ΔΔ G op >7.4 kcal mol −1 ; Supplementary Table S1 ), because it significantly exceeds 6.0 kcal mol −1 . Apparently, exchange of the backbone amide of Ala18 happens less frequently from apoprotein that is temporarily formed on release of FMN from flavodoxin, than occurs from equilibrated apoflavodoxin. We propose that Ala18 is involved in slow structural rearrangements that lead to relaxation of apoflavodoxin after release of FMN. Intermediate stability increases, with ΔΔ G op ranging in between 0.5 to 5.0 kcal mol −1 , occur for 43 residues (coloured green and yellow in Fig. 7 ). Because of the stabilizing effects that FMN imposes, the corresponding opening processes happen less frequently than in apoflavodoxin, but more often than release of FMN from holoprotein takes place. For most residues that are directly involved in intramolecular interactions with FMN, no H/D exchange rates could be measured in apoflavodoxin ( Fig. 6a ; Supplementary Table S1 ) and thus no ΔΔ G op -values were determined. H/D exchange of these residues in apoflavodoxin was not detected, because dynamic exchange of the flavin-binding site between different conformations on the micro- to milli-second timescale causes many of the corresponding NMR cross-peaks to broaden beyond detection [34] . Eighteen of these residues have Δ G op -values in holoprotein of less than 5 kcal mol −1 ( Fig. 6c ; Supplementary Table S1 ), which is significantly less than the free energy associated with FMN release from flavodoxin, as dictated by equation (1). Hence, exchange of these residues happens more frequently than release of FMN from holoprotein and consequently involves small-scale openings of flavodoxin. Rate constants for opening diminish on cofactor binding Cofactor-induced stabilization of amino-acid residues against exposure to solvent can either be achieved by reducing the opening (unfolding) rate of the corresponding protein structure or by accelerating its closing (folding) rate. In case of flavodoxin, 11 residues are identified for which log( k ex ) has a curved dependency on pD in the pD-range used (that is, pD 6.2 to 8.8). For these residues, the equation shown in Fig. 5a is used to fit these data ( Supplementary Methods ). This procedure enables determination of rate constants for opening and closing of the corresponding residues ( Supplementary Table S2 ), with Thr56 as example ( Fig. 5b ). For five residues (that is, Phe6, Ile51, Leu52, Gly53 and Phe94), the rate constants for opening and closing are known for apoprotein as well ( Supplementary Table S2 ). On FMN binding, closing rates reduce 3-to-15 fold, whereas opening rates of these 5 residues reduce about 5,650-fold. Consequently, cofactor binding mainly affects opening events of this FMN-binding protein. Opening rate of flavodoxin's flavin-binding site To follow opening events of the flavin-binding site of flavodoxin, the N(3)H proton of FMN ( Fig. 8a ) is an excellent probe, because its exchange with a deuteron of D 2 O can be measured. To quantitatively interpret H/D exchange of N(3)H, one requires knowledge about whether EX1 or EX2 conditions apply. To distinguish between both situations, we determined the intrinsic rate constant for exchange of N(3)H of FMN free in solution (that is, k int (N(3)H)), which was unknown. The activation energy of exchange for N(3)H is (13.7±1.1) kcal mol −1 , and the intrinsic exchange rate of N(3)H at pD 6.3, 25 °C is (6±2)·10 3 s −1 ( Methods ). 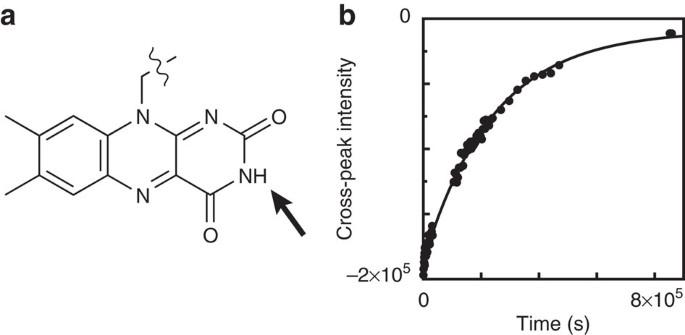Figure 8: Hydrogen exchange of N(3)H of flavodoxin's cofactor. (a) Structure of FMN, with N(3)H indicated. (b) H/D exchange curve obtained for N(3)H of flavodoxin at pD 6.3, 25 °C. Because of folding in the15N-dimension of the1H-15N HSQC experiment, this intensity is negative. The exchange rate is (3.803±0.007)·10−6s−1. Figure 8: Hydrogen exchange of N(3)H of flavodoxin's cofactor. ( a ) Structure of FMN, with N(3)H indicated. ( b ) H/D exchange curve obtained for N(3)H of flavodoxin at pD 6.3, 25 °C. Because of folding in the 15 N-dimension of the 1 H- 15 N HSQC experiment, this intensity is negative. The exchange rate is (3.803±0.007)·10 −6 s −1 . Full size image The exchange rate of the N(3)H proton of FMN in flavodoxin is (3.803±0.007)·10 −6 s −1 at pD 6.3 and 25 °C ( Fig. 8b ). As the corresponding k int (N(3)H) is large (that is, 6×10 3 s −1 ), we expect that N(3)H in flavodoxin exchanges according to the EX1 mechanism. For EX1 conditions to apply, the closing rate k cl of the microenvironment that surrounds N(3)H in flavodoxin needs to be much smaller than k int (N(3)H). This closing reaction is due to binding of FMN to apoflavodoxin and/or due to folding of the microenvironment surrounding N(3)H. Both processes proceed much slower than 6×10 3 s −1 , as the following observations support. First, the rate of binding of FMN to apoflavodoxin is smaller than 1 s −1 (calculated using concentrations of both apoflavodoxin as well as free FMN of about 0.1 μM in a 2.75-mM flavodoxin-containing hydrogen exchange sample, and using a rate constant for binding of FMN [31] of about 1 μM −1 s −1 ). Second, the rate constants for closing of flavodoxin ( Supplementary Table S2 ) and of apoflavodoxin [33] are well below 6×10 3 s −1 . Thus, exchange of N(3)H of flavodoxin indeed occurs according to the EX1 mechanism, and consequently at pD 6.3 and 25 °C the opening rate of flavodoxin's flavin-binding site is (3.803±0.007)·10 −6 s −1 . This paper provides new insights into cofactor-binding interactions. We show by using a well-established titration procedure that the dissociation constant of flavodoxin is 3.51×10 −10 M ( Fig. 1a ). After each titration step, part of the free FMN binds rapidly to apoflavodoxin, causing the associated FMN fluorescence to be quenched nearly instantaneously to low level. This study reveals for the first time that the used titration procedure underestimates the K D -value of cofactor-bound protein, because after this initial quenching extremely slow conformational events happen. Reconstituted holoprotein relaxes with a time constant of ~5 days ( Fig. 2b ) to a state that binds the flavin cofactor about two orders of magnitude better than freshly formed flavodoxin. Many residues are involved in this relaxation process ( Fig. 3 ). Several backbone amide cross-peaks shift with a time constant similar to the one observed by fluorescence, whereas some move more slowly. Apparently, the latter relaxation phenomena do not affect FMN fluorescence. Relaxed flavodoxin is characterized by virtually no fluorescence of bound FMN ( Fig. 2a ) and has a K D of 3.82×10 −12 M ( Fig. 1b ). Thus, tightening of FMN binding leads to an energetically highly favourable protein state with picomolar-binding affinity. Intrinsic exchange of N(3)H in free FMN is about three orders of magnitude faster than intrinsic exchange of backbone amides (that is, k int (N(3)H) equals 6×10 3 s −1 , at pD 6.3 and 25 °C). The corresponding activation energy is 13.7 kcal mol −1 , much less than the 17 kcal mol −1 required for backbone amide exchange [40] . This difference is due to the molecular structure of FMN in which N(3)H is chemically attached to two carbonyl groups ( Fig. 8a ), whereas a backbone amide is coupled to only one carbonyl. Consequently, above pD 6, exchange of N(3)H of protein-bound flavin occurs according to the EX1 mechanism and is an excellent probe to directly measure opening rates of flavin-binding sites. In flavodoxin, N(3)H of FMN is tremendously shielded from solvent. Compared with free FMN, exchange of N(3)H is slowed down by a factor of 1.6×10 9 and thus is a rare event. Each opening event that makes N(3)H accessible to D 2 O causes exchange to occur, because the EX1 mechanism applies. The rate constant of FMN dissociation from flavodoxin is 1.05×10 −6 s −1 ( Fig. 1b ). Hence, H/D exchange of N(3)H occurs (3.6±0.1) times faster than full release of FMN dictates. Consequently, small-scale opening of the microenvironment surrounding N(3)H without dissociation of FMN from the protein must occur, and is in fact the main contributor to this exchange. After nascent apoflavodoxin is released from a ribosome, the protein can autonomously fold to its native state [30] , [31] , [32] , [33] . During apoflavodoxin folding, no transmission of FMN-binding effects happens, because neither unfolded protein nor apoflavodoxin's folding intermediates interact with FMN [31] . Native apoflavodoxin binds to FMN firmly. Under reducing conditions, which prevail in the cytoplasm, tightening of cofactor binding happens rapidly. Because protein-cofactor interactions strongly affect the redox potentials of FMN [16] , [17] , [18] , and because the function-altering amino-acid residues have been evolutionarily selected to optimize protein function, flavodoxin can transfer electrons between various physiological redox partners. We report here the subtle interplay between a protein and its cofactor. By following NMR chemical shifts of backbone amides after reconstitution of flavodoxin, we identified amino-acid residues that tighten cofactor binding from nanomolar to picomolar affinity. By using H/D exchange and NMR spectroscopy, we probed the local free energy differences between apoflavodoxin and fully relaxed flavodoxin and pinpointed amino acids that cause picomolar-binding affinity of the cofactor. Both experiments show that the flavodoxin sequence has evolved such that cofactor-induced effects on local structure and stability not only occur adjacent to FMN, but also happen in many other regions, including distal residues positioned in the core and at the periphery of the protein ( Figs 3 and 7 ). By means of interaction networks, FMN-induced stabilization transmits throughout the entire protein. These networks within apoflavodoxin and flavodoxin comprise hydrogen bonds of α-helices and of the parallel β-sheet, and also involve other intramolecular interactions. From a statistical thermodynamic point of view, the binding of FMN leads to a redistribution of the native-state ensemble. Those states that bind to the cofactor are stabilized with respect to those states that do not, causing a change in the probability distribution of states [10] , [11] . This redistribution affects not only residues in direct contact with FMN, but also regions linked by cooperative interaction networks. Conversely, but fully equivalently, these networks of interacting amino-acid residues cooperate to firmly bind to FMN. Hydrogen exchange of ten residues, coloured orange and red in Fig. 7 , reports the FMN-induced global stability increase. Thus, residues that stabilize the interaction networks and cause tight binding of FMN to flavodoxin have now been experimentally identified for the first time. Because many more amino acids are evolutionarily conserved among flavodoxins, use of alignment of flavodoxin sequences cannot reveal these residues. Two of the residues we identified (that is, Gly8 and Tyr102) are in close contact with FMN. The other eight amino-acid residues (that is, Ala92, Gly95, Asp143, Phe146, Val147, Gly148, Ala150 and Leu151) are far from the flavin. They are dispersed throughout flavodoxin, seem irrelevant to its function, and exert long-range stabilization effects on flavin binding. This study shows that use of NMR spectroscopy and H/D exchange can identify amino-acid residues that cause, by means of interaction networks, the ultimate tight binding of a ligand. Experimental identification of these residues not only is required to understand the thermodynamics of ligand binding, but also is important for engineering, designing and evolving ligand-binding proteins. We show that the interaction between protein and its ligand is complex, and that slow relaxation of flavodoxin happens subsequent to initial binding of FMN. Similar relaxation phenomena are likely relevant for other ligand-binding proteins as well. Ultimately, many residues dispersed throughout the flavodoxin structure contribute to picomolar-binding affinity of FMN. Protein purification The single cysteine at position 69 in wild-type A. vinelandii (strain ATCC 478) flavodoxin II was replaced by an alanine to avoid covalent dimerization of apoflavodoxin. This protein variant is largely similar to wild-type flavodoxin regarding both redox potential of holoprotein and stability of apoprotein [41] , [42] . Uniformly 15 N-labelled recombinant C69A A. vinelandii flavodoxin was obtained from transformed Escherichia coli cells and purified [41] , [42] . This protein contains uniformly 15 N-labelled FMN. Subsequently, apoflavodoxin was prepared using trichloroacetic acid (TCA) as described [30] , [43] . Fluorescence spectroscopy FMN fluorescence was recorded at 25 °C by using a Cary eclipse fluorimeter. FMN was obtained during the TCA-induced preparation of apoflavodoxin and further purified by reverse-phase high-performance liquid chromatography. During the titration procedure, excitation was at 445 nm with a slit of 5 nm and emission was recorded at 525 nm with a slit of 10 nm. During the dilution procedure, excitation was set to 450 nm. A sample of 50 nM FMN was used to correct for photobleaching and instrumental drift. NMR spectroscopy and hydrogen exchange data analysis Lyophilized protein was dissolved in 100 mM potassium pyrophosphate in D 2 O with 100 μM 2,2 dimethyl-2-silapentane-5-sulfonic acid as internal chemical shift reference. The final concentrations of protein ranged in between 1.3 to 3 mM. Samples were immediately transferred into a 500 MHz NMR instrument. Subsequently, a series of HSQC spectra was recorded to detect H/D exchange. The temperature was set to 25 °C. The dead time (that is, the difference in time between mixing D 2 O with lyophilized protein and recording of the first HSQC spectrum) was ~5 min. During H/D exchange, one-dimensional proton NMR spectra of the sample were also acquired. The intensities of the aliphatic resonances in these proton NMR spectra do not alter throughout the course of measuring the series of HSQC spectra. This observation shows unaltered sensitivity of the NMR spectrometer and integrity of the protein sample during our experiments. pD was measured after exchange experiments. Spectra were processed and maximal cross-peak intensities were analysed as a function of time, according to well-established procedures to obtain k ex ( Supplementary Methods ). Rate and equilibrium constants for FMN dissociation The increase in flavin fluorescence due to FMN release when flavodoxin was diluted in buffer was followed at 25 °C. On dilution, the following equilibrium is affected: Return to equilibrium proceeds exponentially as function of time, as it is a first-order process, and the corresponding relaxation time informs about k off as well as K D . Intrinsic rate constant for exchange of N(3)H of FMN In buffer solution, the chemical shift of N(3)H of free FMN can be observed in a 1 H NMR spectrum when the temperature of the sample is set low, to diminish exchange of this rapidly exchanging proton. In addition, one needs a jump-return sequence [44] to avoid excitation of H 2 O and subsequent transfer of saturation to N(3)H. At pH 5.22 and 1.02 °C, N(3)H of free FMN resonates at 11.6 p.p.m. At pD 6.26 and 25 °C, the conditions at which flavodoxin is probed by hydrogen exchange, intrinsic exchange of N(3)H is too rapid to measure directly by NMR spectroscopy. However, the corresponding rate constant k int (N(3)H) can be derived indirectly. A selective saturation recovery NMR experiment [45] , [46] was used to determine k int (N(3)H) at 1.02 °C (verified using 4% methanol in d 4 -methanol) and pH-values of 4.27, 4.72 and 5.22, respectively ( Supplementary Fig. S3 ). FMN concentrations were 100 μM at pH 4.27 and 4.72, and 939 μM at pH 5.22, respectively. Buffer was 100 mM KPPi, 90% H 2 0/10% D 2 O. Fitting of a linear equation to log( k ex ) versus pH shows that the corresponding slope is 0.93±0.13, which equals unity within error ( Supplementary Fig. S3 ). Consequently, in the pH region investigated, exchange of N(3)H is due to catalysis by OH − . To obtain k int (N(3)H) in D 2 O, one needs to take into account the difference in ionization constants of H 2 O and D 2 O, as well as the difference in activities of OH − and OD − (ref. 47 ). In 100 mM KPPi, the activity of OH − at pH 5.65 equals the activity of OD − at pD 6.26. Thus, at pH 5.65 and 1.02 °C, the intrinsic exchange rate of N(3)H is (800±108) s −1 . To extrapolate k int (N(3)H) to 25 °C, the activation energy of exchange ( E a ) for N(3)H needs to be known. To obtain this latter value, a selective saturation NMR experiment was done at 24.53 °C using a solution of 1 mM FMN in 100 mM KPPi pH 4.26. Using these conditions, k ex is (287.9±22.4) s −1 . However, at 1.02 °C, pH 4.27, k ex is (39.6±3.2) s −1 . Using equation 3, the activation energy of exchange for N(3)H was calculated to be (13.67±1.10) kcal mol −1 : with R the gas constant (1.987×10 −3 kcal K −1 mol −1 ). Using the above results, the intrinsic exchange rate of N(3)H at 25 °C and pH 5.65 was inferred to be (6±2)10 3 s −1 . As discussed, this rate also applies at pD 6.26, 25°C, the condition at which the Δ G op -values of the backbone amides of flavodoxin are determined. As mentioned, a selective saturation NMR experiment was used to determine the intrinsic exchange of N(3)H. In this experiment, the pulse sequence (relaxation delay—saturation pulse—variable delay—observation pulse) n was used to determine the apparent longitudinal relaxation rate ( 1 / T 1, app ) of N(3)H, where n is the number of scans acquired. The saturation pulse of 0.15 s was at the frequency of N(3)H and was of sufficient power to saturate this proton. A relaxation delay of 0.5 s was used. During the variable delay period, which ranged from 4 μs to 170 ms, recovery of magnetization of N(3)H occurs. This magnetization was subsequently detected by employing an observation pulse and used to derive T 1,app . A jump-return sequence [44] was used as observation pulse to avoid excitation of H 2 O. In a separate experiment, the H 2 O resonance was saturated during a period of 2.5 s, and subsequently a jump-return sequence was used to detect intensity M s of the N(3)H resonance. In a control experiment, pre-irradiation occurred in an empty region of the spectrum, far removed from both water and N(3)H resonances, to determine intensity M 0 of the N(3)H resonance. Subsequently, the intrinsic rate constant for exchange (1/ τ ) of N(3)H was calculated using [46] : M s turned out to be zero under all experimental circumstances investigated by us and consequently: How to cite this article: Bollen, Y.J.M. et al . Distant residues mediate picomolar-binding affinity of a protein cofactor. Nat. Commun. 3:1010 doi: 10.1038/ncomms2010 (2012).